Female-specific myoinhibitory peptide neurons regulate mating receptivity inDrosophila melanogaster 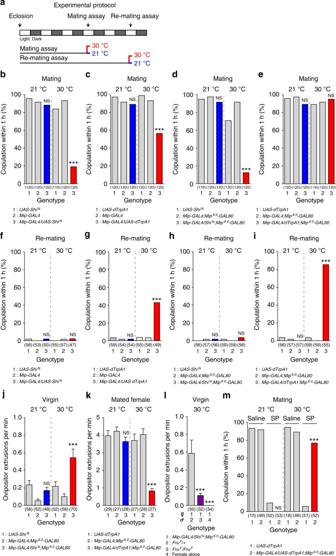Fig. 1 Mip-GAL4neurons switch the mating decision.aThe experimental procedure used for the behaviour assays. Female flies were incubated at the indicated temperatures for 30 min prior to the mating or re-mating assays. For the re-mating assay, females were mated individually with naiveCSmales and kept at 23 °C for 48 h before being paired with a second naiveCSmale.b–eMating frequencies of virgin females of the indicated genotypes, scored as the percentage of females that copulate within 1 h.f–iRe-mating frequencies of mated females.j–lOvipositor extrusions per minute observed in virgin femalesj,lor mated femaleskpaired with naiveCSmalesj,k, males of the indicated genotype or no malel.mMating frequencies of virgin females of the indicated genotypes injected with 12 pmol of sex peptide (SP) in saline or saline alone 2 h prior to the assay. The numbers in parentheses representn. NS indicates non-significance (P> 0.05); ***P <0.001 for comparisons against both controls (grey bars); Chi-square testb–i,mor one-way ANOVA with Tukey’s multiple comparison testj–l. Error bars inj–lindicate s.e.m. Upon mating, fruit fly females become refractory to further mating for several days. An ejaculate protein called sex peptide (SP) acts on uterine neurons to trigger this behavioural change, but it is still unclear how the SP signal modifies the mating decision. Here we describe two groups of female-specific local interneurons that are important for this process—the ventral abdominal lateral ( vAL ) and ventral abdominal medial ( vAM ) interneurons. Both vAL and vAM express myoinhibitory peptide ( Mip ) -GAL4 . vAL is positive for Mip neuropeptides and the sex-determining transcriptional factor doublesex . Silencing the Mip neurons in females induces active rejection of male courtship attempts, whereas activation of the Mip neurons makes even mated females receptive to re-mating. vAL and vAM are located in the abdominal ganglion (AG) where they relay the SP signal to other AG neurons that project to the brain. Mip neuropeptides appear to promote mating receptivity both in virgins and mated females, although it is dispensable for normal mating in virgin females. Depending on environmental and physiological conditions, animals often need to respond differently to the same stimulus. Such behavioural switching is made possible by functional reconfigurations of existing neural circuits. Even the circuits that drive innate behaviours can undergo such reconfigurations [1] . The postmating responses (PMR) of female Drosophila melanogaster are a clear example of this [2] . Prior to mating, female Drosophila accept the courtship advances of males. After mating, however, they actively reject courtship. This suggests the neural circuits that regulate female mating receptivity can exist in at least two distinct functional states, receptive and non-receptive. PMR have emerged as an important behavioural model in which to study the neural processes that reconfigure the functional state of neural circuits in a stable but reversible manner [3] . PMR is induced chemically by a male seminal protein called sex peptide (SP) [4] , [5] . During copulation, the male transfers SP along with sperm into the female uterus [6] , [7] . SP activates SP receptor (SPR) in a small number of SPR-positive sensory neurons (SPSNs), which innervate the uterine lumen and send afferent processes into the tip of the abdominal ganglion (AG) [8] , [9] , [10] , [11] . After the SPSNs, the SP signal is relayed to higher brain areas by two or three SP abdominal ganglion (SAG) neurons, which extensively innervate the AG and project into the dorsal protocerebrum [12] . The SP and SPR pathway seems inhibitory and it signals the postmating state by silencing the SPSNs and SAG neurons [9] , [12] . Silencing the SPSNs or SAGs renders the virgin females unreceptive to mating, while forced activation of the SAGs overrides the SPSN silencing and makes the females regain mating receptivity [12] . Although the SPSN−SAG circuit explains the route by which the peripheral SP signal enters the central nervous system (CNS), the neural and molecular mechanisms that reconfigure the state of the brain and maintain receptivity remain unclear [13] . Neuromodulators like monoamines and neuropeptides change the properties of neural circuits by altering neuronal excitability through slow-acting metabotropic receptors [14] . Decision-making circuits and pattern generators are often multifunctional, with their properties being reconfigured by neuromodulators [15] . In the mammalian thalamus, for example, a cocktail of modulatory substances mediates a switch in the firing pattern of neurons associated with the sleep–wake transition [16] . Likewise, we hypothesize that modulatory substances reconfigure the female mating circuits. Several neuromodulators have already been linked to reproductive behaviours in insects. For example, octopamine has long been implicated in sperm storage, mating and egg laying [17] , [18] , [19] , [20] , [21] . Neurons expressing the neuropeptide SIFamide are associated with female hyper-receptivity [22] . Still, the roles neuromodulators and the neurons that produce them play in female mating behaviours remain largely unexplored [23] . Here we identify two groups of female-specific local interneurons that relay the SP signal from the SPSNs to the SAG neurons and show that a neuropeptide myoinhibitory peptide (Mip) expressed in some of these neurons promotes mating receptivity in females. Screen for postmating switch neurons To identify CNS neurons that modulate female mating decisions, we performed a genetic screen to acutely manipulate the activity of groups of specific neuromodulator neurons in the fly brain and examine the effects on PMR. We used a panel of neuromodulator-specific GAL4 lines to drive the expression of Drosophila transient receptor potential A1 (dTrpA1) or temperature-sensitive shibire (Shi ts ) to temporarily activate or silence (respectively) groups of neurons with a simple temperature shift [24] , [25] . For behavioural assays, we mated individual virgin females carrying either one or two transgenes ( GAL4 and UAS ) to a naive Canton-S ( CS ) male and then tested for receptivity with a second naive CS male 48 h later (re-mating assay). We induced neuronal silencing or activation by shifting the flies to the restrictive temperature (30 °C) shortly after they mated with the first male (Supplementary Fig. 1a ). Of the 39 GAL4 lines we screened, 5 exhibited substantial differences when tested at restrictive vs. permissive temperatures (Supplementary Fig. 1a ). However, of these five, only two lines— Mip-GAL4 line and the Diuretic hormone 44 ( Dh44 )- GAL4 line—continued to exhibit significant differences when compared to the appropriate genetic controls (Supplementary Fig. 1b–f ). Here we focused our analysis on Mip-GAL4 , which produces the strongest mating and re-mating phenotypes. Mip-GAL4 neurons switch the mating decision Previously, we reported the expression of Mip-GAL4 in most Mip-positive neurons in the CNS that are labelled by either an anti-Mip antibody or Mip mRNA in situ hybridization [26] . We will, therefore, refer to Mip-GAL4 neurons as Mip neurons. In our initial screen, we activated or silenced neurons for ~ 48 h prior to the re-mating assay. To avoid any unexpected anomalies caused by chronic (~ 48 h) neuronal activation or silencing, we shifted females to the restrictive temperature 30 min prior to the re-mating assay (Fig. 1a ). Since Mip neuron activation increases mated female receptivity, we asked whether Mip neuron silencing suppresses virgin female receptivity. This was indeed the case—we found that >80% of females with silenced Mip neurons fail to mate within 1 h ( Mip > Shi ts 30 °C; Fig. 1b ). Next we examined the receptivity of virgin females with activated Mip neurons ( Mip > dTrpA1 , 30 °C). Unexpectedly, Mip neuron activation also moderately suppresses virgin female receptivity (Fig. 1c ). The fact that Mip neuron silencing and activation can both reduce mating receptivity depending on mating status suggests that Mip neurons comprise at least two functionally distinct populations, one that facilitates mating and another that suppresses it. To separate these populations genetically, we prepared additional GAL4 transgenes with various fragments of the 5′-upstream regulatory regions of Mip and screened the resulting flies for lines that recapitulate the mating or/and re-mating phenotypes of Mip-GAL4 neuron activation (Supplementary Fig. 2a–c ). None of the GAL4 lines we tested were able to influence the re-mating of mated females, but thermal activation with Mip 6.0 -GAL4 suppresses the mating receptivity of virgin females. Mip 6.0 -GAL4 carries a 6.0 kb fragment of the 5′-upstream regulatory region, whereas Mip-GAL4 carries 7.2 kb fragment (Supplementary Fig. 2a ). To determine whether Mip 6.0 -GAL4 targets a subset of the Mip-GAL4 neurons responsible for inducing mating refractoriness in virgin females, we generated a Mip 6.0 -GAL80 line and combined it with Mip-GAL4 . In these experiments, GAL80 restricts GAL4 activity to a subset of the Mip neurons. Indeed, Mip 6.0 -GAL80 seems to be expressed in the neurons that when activated suppress mating receptivity, because at 30 °C, Mip 6.0 -GAL80 blocks the suppression of receptivity observed in Mip > dTrpA1 virgin females but not in Mip > Shi ts females (Fig. 1d, e ). Mated flies, however, re-mate more frequently than those lacking Mip 6.0 -GAL80 (Fig. 1g, i ). Mip 6.0 -GAL80 does not affect the phenotypes induced by Mip neuron silencing (Fig. 1f, h ). Fig. 1 Mip-GAL4 neurons switch the mating decision. a The experimental procedure used for the behaviour assays. Female flies were incubated at the indicated temperatures for 30 min prior to the mating or re-mating assays. For the re-mating assay, females were mated individually with naive CS males and kept at 23 °C for 48 h before being paired with a second naive CS male. b – e Mating frequencies of virgin females of the indicated genotypes, scored as the percentage of females that copulate within 1 h. f – i Re-mating frequencies of mated females. j – l Ovipositor extrusions per minute observed in virgin females j , l or mated females k paired with naive CS males j , k , males of the indicated genotype or no male l . m Mating frequencies of virgin females of the indicated genotypes injected with 12 pmol of sex peptide (SP) in saline or saline alone 2 h prior to the assay. The numbers in parentheses represent n . NS indicates non-significance ( P > 0.05); *** P < 0.001 for comparisons against both controls (grey bars); Chi-square test b – i , m or one-way ANOVA with Tukey’s multiple comparison test j–l . Error bars in j–l indicate s.e.m. Full size image Mated females actively reject courting males by forcefully extruding their ovipositors in response to male advances. We examined the effects of Mip neuron activation or silencing on the rejection behaviour while subtracting the Mip 6.0 -GAL80 neurons. We found Mip neuron activation suppresses ovipositor extrusion by 80% (Fig. 1k ), whereas Mip neuron silencing enhances it (Fig. 1j and Supplementary Movie 1 ). To exclude the possibility that the Mip neurons are involved in the motor output required for ovipositor extrusion rather than controlling mating receptivity, we asked whether Mip neuron silencing induces ovipositor extrusion even in the absence of courting males (Fig. 1l ). In Drosophila , the fruitless ( fru ) gene encodes a sexually dimorphic transcription factor that is closely linked to male sexual orientation [27] . Males homozygous for fru F show very little courtship towards females [28] . When paired with fru F /fru F males, virgin females with silenced Mip neurons show no increase in ovipositor extrusion, indicating that the rejection behaviour caused by Mip neuron silencing occurs only in response to male advances. Indeed, ovipositor extrusion never occurs in isolated females. It is important to note that mated control females show ~ 8 times more frequent ovipositor extrusion than virgin females with silenced Mip neurons. This may be due to insufficient Mip neuron silencing or it may indicate additional neural components operating in mated females. Nevertheless, these results suggest the Mip neurons that are not labelled by Mip 6.0 -GAL80 can switch the mating decision on or off regardless of a female’s previous mating experience. Despite robust effects on receptivity, neither activation nor silencing of Mip neurons affects the fecundity of mated females (Supplementary Fig. 3a, b ). In virgin females, however, Mip neuron silencing slightly increases egg laying (Supplementary Fig. 3c ). This is similar to the increase in virgin egg laying induced by silencing the SAG neurons [12] . Mip-GAL4 neurons signal downstream of SP The effects of SP on mating receptivity and egg laying are mediated by SPR expressed in a small subset of uterine fruitless ( fru ), doublesex ( dsx ) and pickpocket ( ppk )-positive SPSNs that arborize in the lumen of the uterus and project to the CNS [9] , [10] , [11] . Their innervation pattern suggests that these neurons detect SP inside the uterus and relay this signal directly into the CNS. We examined female flies expressing dsRed in Mip-GAL4 neurons and enhanced green fluorescent protein (EGFP) in ppk neurons to determine whether SPSNs express Mip-GAL4 . Because there was no Mip-GAL4 -positive process among ppk + SPSNs in the uterus (arrows in Supplementary Fig. 4a ), we explored the possibility that SP directly modulates central Mip neurons. This is important because male-derived SP circulates in the haemolymph of mated females [6] , [29] and SPR is expressed broadly in the CNS [8] . Although Mip neuron-specific knockdown of SPR does not affect PMR, ppk neuron-specific SPR knockdown strongly suppresses PMR, allowing flies to re-mate [9] , [10] (Supplementary Fig. 4b ). Furthermore, SPR expression in ppk neurons but not Mip neurons rescues PMR in SPR mutants (Supplementary Fig. 4c ). These results indicate that SPR expression in Mip neurons is neither necessary nor sufficient to elicit PMR. We next examined the behaviour of flies expressing a membrane-tethered form of SP (mSP) [30] in Mip neurons to test the possibility that SP directly modulates Mip neurons via SPR or a second unidentified SP receptor. As previously reported [9] , virgin females expressing mSP in their ppk neurons are as unreceptive as mated females, but females expressing mSP in Mip neurons are as receptive as wild-type controls (Supplementary Fig. 4d ). We conclude, therefore, that SP does not directly modulate Mip neurons and that Mip neurons constitute a CNS circuit that operates downstream of SP-SPR signalling. To test this, we asked whether Mip neuron activation can override the effects of SP in vivo . We injected virgin females with synthetic SP, which suppresses mating receptivity [4] , [8] , [31] . Thermal activation of Mip neurons makes these SP-injected females as receptive as saline-injected controls (Fig. 1m ). This epistatic effect of Mip neuron activation over SP injection indicates that the Mip neurons function downstream of SP-SPR signalling, presumably as SPSNs. Mip neurons in the CNS Since Mip neurons appear to function downstream of SPSNs, and SPSNs send afferent processes into the AG, we reasoned that the behaviourally relevant Mip neurons reside in the CNS. Thus we examined the expression pattern of Mip-GAL4 , Mip 6.0 -GAL4 and Mip 6.0 -GAL80 in the female CNS (Fig. 2a–c ) using anti-Mip staining as a reference. Although the CNS expression of Mip-GAL4 was previously reported [26] , we included it in our analysis for direct comparisons with other transgenes (Fig. 2a ). As shown previously, Mip-GAL4 is expressed in ~ 230 CNS neurons. Virtually all 52 anti-Mip neurons are positive for Mip-GAL4 , but the converse is not true. Likewise, Mip 6.0 -GAL4 is expressed in most anti-Mip neurons, except for two pairs of superior anterior medial (SAM) neurons and one pair of inferior contralateral interneurons in the brain (in dotted red circles in the cartoon in Fig. 2b ). Mip 6.0 -GAL4 is also expressed in additional neurons lacking anti-Mip staining, which include myriad optic lobe neurons (indicated by green shading in the cartoon in Fig. 2b ), 112 non-optic lobe brain neurons and 56 ventral nerve cord (VNC) neurons. Except for 46 anti-Mip neurons that express both Mip-GAL4 and Mip 6.0 -GAL4 (compare cartoons in Fig. 2a, b ), the both GAL4 neuron populations seem largely different from each other. Lastly, we examined the Mip 6.0 -GAL80 expression using females carrying both the Mip-Gal4 and Mip 6.0 -GAL80 transgenes. 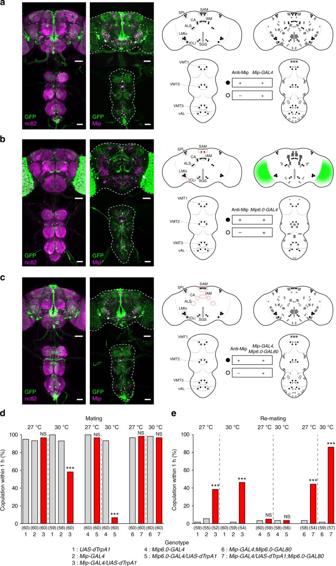Fig. 2 Mip neurons in the CNS.a–cMipneurons in a 4-day-old virgin female bearingaMip-GAL4, UAS-mCD8-EGFP,bMip6.0-GAL4, UAS-mCD8-EGFPandcMip-GAL4, Mip6.0-GAL80, UAS-mCD8-EGFPstained with anti-GFP (green) and anti-nc82 (magenta) or anti-GFP (green) and anti-Mip (magenta) antibodies. The left schematic shows anti-Mip and EGFP-positive neurons (closed circles). The right schematic includes EGFP neurons that lack anti-Mip labelling (open circles). In the left schematic, dotted black circles group anti-Mip neuron classes. Dotted red circles indicate groups that lack complete labelling ofMipneuron(s), compared withMip-GAL4. Green shading in the schematic inbindicates a large number of uncounted EGFP-positive cell bodies.SAMsuperior anterior medial,SPLsuperior posterior lateral,IAMinferior anterior medial,ALSantennal lobe superior,SGSsubesophageal superior,CAcentral anterior,ICLIinferior contralateral interneurons,SGIsubesophageal inferior,LMIolateral MIP-IR optic lobe,VMT1ventral medial thoracic 1,VMT2ventral medial thoracic 2,VMT3ventral medial thoracic 3,vALventral lateral abdominal. Scale bars, 50 μm.dMating frequencies of virgin females of the indicated genotypes, scored as the percentage of females that copulate within 1 h.eRe-mating frequencies of mated females. The numbers in parentheses indicaten. NS indicates non-significance (P> 0.05); ***P< 0.001 for comparisons against both controls (grey bars); Chi-square testd,e Despite the overlap of Mip-GAL4 and Mip 6.0 -GAL4 expression in anti-Mip neurons, Mip 6.0 -GAL80 blocks the Mip-GAL4 expression in few Mip 6.0 -GAL4 -positive brain anti-Mip neurons including the SAM, antennal lobe superior, central anterior and inferior anterior medial neurons (see dotted red circles in the cartoon in Fig. 2c ). Although all anti-Mip neurons in the VNC are positive for both Mip-GAL4 and Mip 6.0 -GAL4 , Mip 6.0 -GAL80 does not block GAL4 activity in any of the VNC neurons. Fig. 2 Mip neurons in the CNS. a – c Mip neurons in a 4-day-old virgin female bearing a Mip-GAL4, UAS-mCD8-EGFP , b Mip 6.0 -GAL4, UAS-mCD8-EGFP and c Mip-GAL4, Mip6.0-GAL80, UAS-mCD8-EGFP stained with anti-GFP (green) and anti-nc82 (magenta) or anti-GFP ( green ) and anti-Mip (magenta) antibodies. The left schematic shows anti-Mip and EGFP-positive neurons (closed circles). The right schematic includes EGFP neurons that lack anti-Mip labelling (open circles). In the left schematic, dotted black circles group anti-Mip neuron classes. Dotted red circles indicate groups that lack complete labelling of Mip neuron(s), compared with Mip-GAL4 . Green shading in the schematic in b indicates a large number of uncounted EGFP-positive cell bodies. SAM superior anterior medial, SPL superior posterior lateral, IAM inferior anterior medial, ALS antennal lobe superior, SGS subesophageal superior, CA central anterior, ICLI inferior contralateral interneurons, SGI subesophageal inferior, LMIo lateral MIP-IR optic lobe, VMT1 ventral medial thoracic 1, VMT2 ventral medial thoracic 2, VMT3 ventral medial thoracic 3, vAL ventral lateral abdominal. Scale bars, 50 μm. d Mating frequencies of virgin females of the indicated genotypes, scored as the percentage of females that copulate within 1 h. e Re-mating frequencies of mated females. The numbers in parentheses indicate n . NS indicates non-significance ( P > 0.05); *** P < 0.001 for comparisons against both controls (grey bars); Chi-square test d , e Full size image Optimization of dTrpA1-mediated Mip neuron activation The population of Mip-GAL4 neurons seems to be composed of at least two functionally opposing subsets: dTrpA1-mediated activation of one subset suppresses mating, while activation of the other promotes mating. We suspected that these subsets may have different temperature requirements for thermal activation. If so, we hoped to be able to activate one subset without activating the other simply by optimizing the activation temperature. Indeed, incubation at 27 °C does not suppress the virgin mating receptivity of Mip > dTrpA1 females, but still increases re-mating by ~ 40% (Fig. 2d, e ). Consistent with this result, Mip 6.0 -GAL4 neurons expressing dTrpA1 have little impact on mating receptivity at 27 °C but almost completely suppress mating receptivity at 30 °C. Activation of the mating promoting subset alone ( Mip-GAL4 , Mip 6.0 -GAL80 , UAS-dTrpA1 ) increases re-mating by ~ 40% at 27 °C and almost fully at 30 °C. Together, these observations indicate that a 27 °C incubation at least partially activates the pro-mating circuit without activating the antimating circuit in Mip > dTrpA1 females. Mip is involved in female mating receptivity We previously generated a Mip-null allele ( Mip 1 ) in which the entire Mip coding sequence is replaced by the mini-white gene [26] . When paired with naive CS males, Mip-deficient virgin females ( Mip 1/1 ) mate normally (Fig. 3a ). We previously observed that knockdown of Mip across the nervous system does not affect the receptivity of either virgin or mated females [32] . Next, we examined re-mating of mated Mip 1/1 females while activating their Mip neurons. Thermal activation of Mip neurons does increase re-mating in the Mip mutant background but not nearly as much as in the presence of the wild-type Mip allele (Fig. 3b ). Although this experiment indicates that Mip promotes re-mating, neither Mip overexpression in the Mip neurons ( Mip > Mip ) nor in the entire nervous system ( elav > Mip ) affects mating latency in virgins or re-mating frequency in mated females (Fig. 3c, d , respectively). Fig. 3 A function of Mip peptides in female mating receptivity. a Mating frequencies of virgin females of the indicated genotypes, scored as the percentage of females that copulate within 1 h. b , d Re-mating frequencies of mated females. NS indicates non-significance ( P > 0.05); *** P < 0.001 for comparisons against controls; Chi-square test a , b , d . c , e , f Cumulative mating frequencies of virgin females. The numbers in parentheses indicate n . NS indicates non-significance ( P > 0.05); *** P < 0.001 for comparisons against genetic controls (grey bars or dots in a – d ) or a temperature control (blue in e , f ); Chi-square test Full size image The Mip gene encodes several closely related Mip neuropeptides, which are highly selective and potent agonists of SPR [32] , [33] . Thus it seems likely that Mip neuron activation induces the secretion of Mip peptides, which, in turn, activate SPR and suppress mating receptivity. Unexpectedly, however, we found that Mip neuron activation increases the sexual receptiveness of mated females, partly through Mip gene products (Fig. 3b ). It, therefore, seems unlikely that Mip acts through SPR to promote re-mating. To test this directly, we wanted to examine re-mating in SPR-deficient females while activating their Mip neurons. Unfortunately, this experiment is impossible; SPR-deficient females are sexually receptive regardless of mating status. Instead, we asked whether Mip neuron activation facilitates the first mating event and then whether its enhancement of mating persists in the absence of Mip or SPR (Fig. 3e, f , respectively). We first compared the cumulative mating of Mip > dTrpA1 virgin females paired with CS males at 21 and 27 °C. We used 27 °C for thermal activation to minimize the activation of the subpopulation of Mip neurons that inhibits mating (i.e., those that express Mip 6.0 -GAL4 , see Fig. 2d, e ). Virgin females whose Mip neurons are activated at 27 °C engage in their first mating more rapidly than controls incubated at 21 °C (Fig. 3e ). Subsequently, we examined Mip > dTrpA1 and its controls in the Mip - and SPR -deficient backgrounds. As expected, Mip neuron activation does not promote mating in females that lack Mip (Fig. 3e ). Surprisingly, the loss of SPR does not affect the increase in mating induced by Mip neuron activation (Fig. 3f ). These results strongly suggest that the effects of Mip on mating are mediated by a receptor other than SPR. Dsx + abdominal Mip neurons control female receptivity Mip-GAL4 is expressed mainly in the central neurons of the brain and VNC [26] . To map the Mip neurons that are functionally relevant to mating behaviour, we examined the Mip neurons that express fruitless ( fru ) or doublesex ( dsx ) because these genes are causally linked to several gender-specific behaviours [21] , [34] , [35] , [36] , [37] , [38] . We previously reported that a small number of brain Mip neurons are positive for fru FLP (Supplementary Fig. 5a ) [26] . Neither silencing nor activating these Mip and fru FLP double-positive central neurons affects female mating receptivity (Supplementary Fig. 5b, c ). In contrast, silencing Mip and dsx FLP double-positive neurons (hereafter Mip/dsx ) markedly suppresses virgin receptivity (Fig. 4a ), although their thermal activation does not increase re-mating in mated females (Fig. 4b ). We next examined EGFP-labelled Mip/dsx neurons in the CNS of females carrying Mip-GAL4 , UAS-FRT-stop cassette-FRT-mCD8-EGFP and either one or two copies of the dsx FLP transgene (Fig. 4c, d ). After noting more reproducible labelling of Mip/dsx neurons in females carrying two copies of dsx FLP , we detected two pairs of Mip/dsx neurons in the brain and two pairs in the AG (Fig. 4c, d ). To separate the functions of these neurons, we added an otd FLP transgene, which is active exclusively in the brain, not the VNC (Supplementary Fig. 5d ) [39] . Neither silencing nor activating the Mip/otd neurons affects mating in virgin or mated females (Supplementary Fig. 5e, f ). This suggests it is unlikely that the brain Mip neurons are involved. Thus we concluded that Mip/dsx neurons in the AG constitute a part of the neural circuit that, when active, maintains female sexual receptivity. The Mip/dsx neurons in the AG are also stained by the anti-Mip antibody (Fig. 4e , upper panel). Based on the location of their somas, we propose naming them ventral anterior lateral neurons of the AG (hereafter vAL ). The anatomy of the vAL neurons suggests they are local interneurons that extensively innervate the AG and project to the meso-thoracic ganglion along the midline (Fig. 4e , lower panel). We next defined the input and output domains of vAL by driving expression of the postsynaptic marker nSyb and the presynaptic marker Dscam, respectively. We found that the vAL neurons appear to receive inputs from the abdomen and send outputs to both the abdomen and thorax via processes that run along the midline (Fig. 4f, g ). Fig. 4 Doublesex -positive abdominal Mip neurons are important for female receptivity. a Mating frequencies of virgin females of the indicated genotypes, scored as the percentage of females that copulate within 1 h. b Re-mating frequencies of the mated females. The numbers in parentheses indicate n . NS indicates non-significance ( P > 0.05); *** P < 0.001 for comparisons against both controls (grey bars); Chi-square test a , b . c Mip and dsx double-positive neurons in a female carrying Mip-GAL4, UAS > stop > mCD8-GFP and two copies of dsx FLP stained with anti-GFP (green) and anti-nc82 (magenta) antibodies. d The number of GFP-positive soma in the brain and VNC from females of the indicated genotypes. *** P < 0.001; unpaired t -test. Error bars indicate s.e.m. e Mip and dsx double-positive vAL neurons in the AG of a female carrying Mip-GAL4 , UAS > stop > mCD8-GFP and one copy of dsx FLP stained with anti-GFP (green) and anti-Mip (magenta) antibodies (upper panel). Note that only one of the four vAL neurons stained in the AG of this specific preparation with the anti-Mip (magenta) antibody is GFP-positive (green). The lower panel is a negative image of the green channel from the upper panel image. Note that the single vAL cell extensively innervates the AG and projects one afferent axon along the midline to the thoracic ganglion. f vAL neurons from a female carrying Mip-GAL4 , UAS > stop > nSyb-GFP and dsx FLP stained with anti-GFP (green) and anti-nc82 (magenta). Note the localization of the presynaptic marker nSyb-GFP along the midline of the TG as well as in the AG. g vAL neurons from a female carrying Mip-GAL4 , UAS > stop > Dscam-GFP and dsx FLP stained with anti-GFP (green) and anti-nc82 (magenta). h A high magnification view of the AG from a female carrying Mip-GAL4 , UAS > stop > nSyb-GFP and dsx FLP stained with anti-GFP (green) and anti-Mip (magenta). Arrowheads indicate vAL somas h – k . i The AG from a female carrying Mip-GAL4 , UAS > stop > Dscam-GFP and dsx FLP stained with anti-GFP (green) and anti-Mip (magenta). j The AG from a female carrying SPSN-GAL4 and UAS-mCD8-EGFP stained with anti-GFP (green) and anti-Mip (magenta). k The AG from a female carrying SAG-GAL4 and UAS-mCD8-EGFP stained with anti-GFP (green) and anti-Mip (magenta). All scale bars, 50 μm Full size image vAL neurons intermingle with SPSN and SAG neurons The SPSN neurons that detect SP in male ejaculate send their axon terminals to the tip of the AG. Because vAL neurons are the only Mip-positive neurons in the AG and because the anti-Mip staining in the AG co-localizes with both nSyb and Dscam (Fig. 4h, i ), we suspected we could use anti-Mip staining of SPSN neural processes in the AG to visualize anatomical interactions between vAL and SPSNs. As expected, we observed intermingling of anti-Mip staining with SPSN processes in the AG (Fig. 4j ). Likewise, we also noted anatomical interactions between vAL neurons and the SAG neurons that project to higher brain areas (Fig. 4k ) [12] . Female-specific Mip neurons in the AG Successful mating requires gender-specific neural processing. Thus we compared Mip neurons in males and females. Since the brain Mip neurons are likely irrelevant, we focussed our analysis on the VNC neurons. We found clear sexual dimorphism in the Mip neurons of the AG. The abdominal Mip neurons labelled with Mip-GAL4 , Mip 6.0 -GAL80 and UAS-mCD8-EGFP in females are divided into five groups according to the relative locations of their somas (Fig. 5a ): the anti-Mip and dsx -positive vAL , ventral anterior medial ( vAM ), small ventral posterior medial ( s-vPM ), large ventral posterior medial ( l-vPM ), and small medial posterior medial ( s-mPM ). Apart from vAL , no other AG cells express anti-Mip. In males, we found no labelled neurons in the AG regions where vAL and vAM neurons are in females (Fig. 5a, b ). Fig. 5 Sexually dimorphic Mip neurons in the AG that regulate female receptivity. a Mip neurons in the AG from a female (above left) and a male (above right) carrying Mip-GAL4 , Mip6.0-GAL80 and UAS-mCD8-GFP stained by anti-GFP (green) and anti-nc82 (magenta) antibodies. The lower panels indicate the numbers and relative locations of Mip neuron somas in female (left) and male (right) AGs. The Mip neurons in the AG are grouped into six subsets: medial anterior lateral ( mAL ), ventral anterior lateral ( vAL ), ventral anterior medial ( vAM ), small ventral posterior medial ( s-vPM ), large ventral posterior medial ( l-vPM ), and small medial posterior medial ( s-mPM ). Filled and open circles indicate neurons positive and negative for anti-Mip, repectively. Scale bars, 50 μm. b The numbers of GFP-positive Mip neurons in the AGs of females (green) and males (red) carrying Mip-GAL4 , Mip6.0-GAL80 and UAS-mCD8-EGFP . Note the clear sexual dimorphism in the vAL and vAM neurons. c Negative images of TRIC labelling (anti-GFP) in the AGs of virgin (upper panels) and mated females (lower panels), indicating intracellular Ca 2+ transients. Scale bars, 10 μm. d The GFP intensities from vAM , l-vPM and SAG neurons of TRIC females show Ca 2+ activity in virgin (green) and mated females (red). e The frequencies of labelled (and therefore activated) neurons in the indicated Mip neuron subset of the AG from non-re-mating (green) and re-mating mosaic females (red). We used females carrying hsFLP , Mip-GAL4 , UAS-TrpA1 , UAS-DsRed and Tub FRT GAL80 FRT for stochastic manipulation (for details, see the text). NS indicates non-significance ( P > 0.05); ** P < 0.01, *** P < 0.001. Unpaired t -test for b , d , e . Error bars indicate s.e.m. Full size image Because Mip neuron activation increases re-mating, we reasoned that the relevant Mip neurons would show higher activity levels in virgin females than mated females. We, therefore, asked whether AG neurons change their activity before and after mating. We monitored Mip neuron activity using an end-point Ca 2+ reporting system, the transcriptional reporter of intracellular Ca 2+ (TRIC). TRIC is designed to increase GFP expression in proportion to intracellular Ca 2+ levels [40] . In virgin females, we detected robust TRIC signal in vAM , l-vPM and SAG neurons (Fig. 5c ). We measured the SAG neurons as a positive control. Measuring 48 h after mating, we observed significant attenuation of the TRIC signal intensity in vAM and SAG but not in l-vPM soma (Fig. 5c, d ). This suggests the secretory activities of vAM and SAG are significantly reduced after mating. This is consistent with our behavioural observations; silencing either the vAM or SAG neurons induces strong mating refractoriness, a key feature of PMR. We noted that the TRIC signal changes not only in the soma but also in the neural processes (arrowheads in virgin and mated SAG in Fig. 5c ). No other AG Mip neurons, including l-vPM , show mating-induced TRIC signal changes. In particular, s-vPM and s-mPM show no or very weak TRIC signal regardless of mating status (Supplementary Fig. 6 ). We were unable to detect any TRIC signal in vAL neurons, regardless of mating status (Supplementary Fig. 6 ). This lack of TRIC signal suggests that the activity of vAL neurons differs from that of vAM neurons. 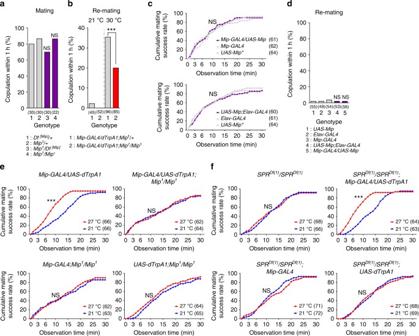Fig. 3 A function of Mip peptides in female mating receptivity.aMating frequencies of virgin females of the indicated genotypes, scored as the percentage of females that copulate within 1 h.b,dRe-mating frequencies of mated females. NS indicates non-significance (P> 0.05); ***P< 0.001 for comparisons against controls; Chi-square testa,b,d.c,e,fCumulative mating frequencies of virgin females. The numbers in parentheses indicaten. NS indicates non-significance (P> 0.05); ***P< 0.001 for comparisons against genetic controls (grey bars or dots ina–d) or a temperature control (blue ine,f); Chi-square test Our finding that vAM activity undergoes a significant switch after mating links these neurons to the control of female mating receptivity. We noted that activation of vAL alone (i.e., dsx FLP -positive Mip-GAL4 neurons) does not induce the re-mating phenotype in mated females, whereas activation of all Mip neurons does. Thus vAM neurons seem to only be partially responsible for the re-mating phenotype. To explore this idea, we adopted a mosaic approach employing an excisable GAL80 [41] . We prepared flies carrying Mip-GAL4 , UAS-dTrpA1 , UAS-dsRed , tubulin-FRT-GAL80-FRT ( tub > GAL80 > ) and the heatshock-flippase ( hs-FLP ). In this system, a brief exposure to high temperature (37 °C, 35 min) induces FLP expression. FLP then excises GAL80 in a small fraction of Mip-GAL4 neurons per fly, permitting dTrpA1 and dsRed expression only in the affected cells. We proceeded to count the dsRed/dTrpA1-positive AG neurons in mosaics with and without the re-mating phenotype when they were incubated at 30 °C. Of the five groups of AG Mip neurons, only the vAM neurons show significantly more dsRed labelling in re-mating mosaics than in non-re-mating mosaics (Fig. 5e ). This suggests that the sexually dimorphic vAM neurons are important for regulating female mating receptivity. Since we do not yet have any genetic tools for isolating vAM neurons at single cell resolution, we were unable to determine where and how they innervate the different parts of the CNS. A careful analysis of their TRIC labelling, however, suggests that vAM neurons are local interneurons with no obvious afferent processes (Supplementary Fig. 6 ). Mip neurons relay the SP signal to SAG neurons Our analyses suggest that the Mip neurons are part of the SPSN–SAG circuit and are likely positioned between the SPSNs and the SAG neurons. This is because Mip -positive vAL neuron silencing abolishes female mating receptivity just like SAG neuron silencing (Fig. 4a ) and because vAL processes intermingle with SPSN and SAG processes without projecting to the brain or uterus themselves (Fig. 4j, k ). To test this model, we looked for functional epistasis. When we silenced either the SPSNs or SAGs with Kir2.1 (SPSN− and SAG−, respectively), we found that virgin females are unreceptive. This is expected because SP activates an inhibitory G-protein coupled receptor (GPCR) SPR in the SPSNs, which upon activation induces PMR by silencing the SPSNs directly and SAG neurons indirectly [8] , [9] , [12] . We next asked whether Mip neuron activation can override this SPSN− condition. Indeed, Mip neuron activation renders virgin females receptive even in the SPSN− condition, indicating that Mip neurons function downstream of SPSNs (Fig. 6a ). In this experiment, we observed only partial restoration of mating receptivity (~ 40%) because Mip-GAL4 targets both mating-promoting neurons (i.e., vAL and vAM ) and mating-suppressing neurons (i.e., those that express Mip 6.0 -GAL4 , see Fig. 2d ). Finally, we asked whether Mip neuron activation restores mating receptivity in the SAG− condition and found that it does not (Fig. 6b ). This is consistent with our model that Mip neurons function upstream of SAGs. Together, these observations suggest that Mip neurons are indeed part of the SPSN–SAG circuit and that they relay the SP signal from SPSNs to SAGs (Fig. 6c ). Fig. 6 Mip neurons positioned within the SPSN and SAG signalling axis. a , b Mating frequencies of virgin females of the indicated genotypes, scored as the percentage of females that copulate within 1 h. The numbers in parentheses indicate n . NS indicates non-significance ( P > 0.05); *** P < 0.001 for comparisons against both controls (grey bars); Chi-square test a , b . c Model explaining the hierarchical relationships of the various components of the AG circuits that control female receptivity (for details, see the text) Full size image To make a mating decision, Drosophila females compute the sensory inputs they receive from courting males and integrate them with the internal state coding SP signals originating in their reproductive organs. An early gynandromorph study [42] mapped this computational function to the brain. More recently, a small number of dsx -positive brain neurons were found to receive courtship-related olfactory and auditory inputs and to regulate female mating [43] . On the other hand, the uterine SP signal is relayed to the central brain through the SPSN–SAG circuit. By combining channelrhodopsin-mediated activation of SPSNs and patch-recording of the SAG neurons, SPSN activation was shown to elicit excitatory postsynaptic potentials (EPSPs) in SAG neurons [12] . Because the average latency from SPSN activation to the corresponding SAG EPSP is ~ 20 ms—far longer than the 1–2 ms expected for a monosynaptic connection—the SPSN–SAG connection is likely polysynaptic. Furthermore, we noted that mating attenuates not only the frequency but also the amplitude of SAG EPSPs triggered by SPSN activations [12] . This amplitude modulation seems to suggest that SAG neurons receive multiple synaptic inputs. It is possible that SPSNs modulate vAM and vAL neurons, which then feed excitatory synaptic inputs to SAG neurons (Fig. 4f ). Consistent with this model, Mip neuron activation overrides SP injection or SPSN silencing but not SAG silencing. This functional epistasis suggests Mip neurons (i.e., vAL and vAM ) function downstream of SPSNs and upstream of SAGs. Because SP can access central neurons via the haemolymph, SP may modulate SAG EPSPs by directly acting on the vAM and vAL neurons. Since Mip neuron-specific mSP expression elicits no sign of PMR-like behaviours, SP actions on those are less likely. Our genetic analyses of the Mip mutants indicate that the Mip neuropeptides can promote mating receptivity both in virgin and mated females. Mip is a potent and physiologically relevant agonist for SPR [32] , [33] . Like other neuromodulators, Mip is highly pleiotropic, being involved in behaviours as diverse as sleep and feeding [26] , [44] . SPR mediates the sleep function of Mip but is dispensable for its feeding function [26] , [44] . Our observation that the mating function of Mip does not require SPR suggests the presence of another unknown Mip receptor (hereafter referred to as hypothetical Mip receptor 1 or hMipR1). The SPSN–SAG circuit fires more frequently in virgin females than in mated females. Since vAL neurons are a part of the SPSN–SAG circuit, they should actively release Mip neuropeptides in virgin females. These, in turn, should activate SPR at the SPSN axon terminals and induce PMR. We found, however, that rather than supressing mating receptivity, hyper-activation of vAL increases it. Why is this? The simplest explanation is that SPR is absent from the SPSN axon terminals exposed to Mip. The subcellular localization of most metabotropic neurotransmitter receptors and other GPCRs is not tightly controlled and many of these proteins show extrasynaptic localization [45] . Alternatively, if Mip activates both SPR and hMipR1 and if they suppress and promote mating receptivity, respectively, the activation of hMipR1 may dominate the effect of SPR activation. 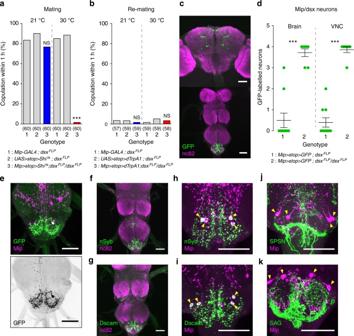Fig. 4 Doublesex-positive abdominalMipneurons are important for female receptivity.aMating frequencies of virgin females of the indicated genotypes, scored as the percentage of females that copulate within 1 h.bRe-mating frequencies of the mated females. The numbers in parentheses indicaten. NS indicates non-significance (P> 0.05); ***P< 0.001 for comparisons against both controls (grey bars); Chi-square testa,b.cMipanddsxdouble-positive neurons in a female carryingMip-GAL4, UAS>stop>mCD8-GFPand two copies ofdsxFLPstained with anti-GFP (green) and anti-nc82 (magenta) antibodies.dThe number of GFP-positive soma in the brain and VNC from females of the indicated genotypes. ***P< 0.001; unpairedt-test. Error bars indicate s.e.m.eMipanddsxdouble-positivevALneurons in the AG of a female carryingMip-GAL4,UAS>stop>mCD8-GFPand one copy ofdsxFLPstained with anti-GFP (green) and anti-Mip (magenta) antibodies (upper panel). Note that only one of the fourvALneurons stained in the AG of this specific preparation with the anti-Mip (magenta) antibody is GFP-positive (green). The lower panel is a negative image of the green channel from the upper panel image. Note that the singlevALcell extensively innervates the AG and projects one afferent axon along the midline to the thoracic ganglion.fvALneurons from a female carryingMip-GAL4,UAS>stop>nSyb-GFPanddsxFLPstained with anti-GFP (green) and anti-nc82 (magenta). Note the localization of the presynaptic marker nSyb-GFP along the midline of the TG as well as in the AG.gvALneurons from a female carryingMip-GAL4,UAS>stop>Dscam-GFPanddsxFLPstained with anti-GFP (green) and anti-nc82 (magenta).hA high magnification view of the AG from a female carryingMip-GAL4,UAS>stop>nSyb-GFPanddsxFLPstained with anti-GFP (green) and anti-Mip (magenta). Arrowheads indicatevALsomash–k.iThe AG from a female carryingMip-GAL4,UAS>stop>Dscam-GFPanddsxFLPstained with anti-GFP (green) and anti-Mip (magenta).jThe AG from a female carryingSPSN-GAL4andUAS-mCD8-EGFPstained with anti-GFP (green) and anti-Mip (magenta).kThe AG from a female carryingSAG-GAL4andUAS-mCD8-EGFPstained with anti-GFP (green) and anti-Mip (magenta). All scale bars, 50 μm SPR deficiency, however, has little impact on the mating induced by Mip neuron activation. This suggests that SPR activation by Mip does not induce PMR-like mating refractoriness. It also suggests that Mip and SP are biased GPCR ligands that recruit different signalling pathways downstream of SPR [46] . We, therefore, propose the following scenario: Activation of vAL neurons produces virgin-like mating receptivity because Mip released from vAL neurons activates hMipR1 in SAG neurons while simultaneously desensitizing SPR locally in SPSN processes that arborize in the AG. vAM neurons also contribute to this process by releasing unknown substances that synergize with the actions of Mip (Fig. 6c ). Fly stocks Fly lines were raised at 25 °C and 60% humidity in 12 h:12 h light:dark cycle with the standard fly media. Following stocks are reported previously or obtained from the Bloomington Drosophila Stock Center (BDSC): Ccap-GAL4 [47] , AstCC-GAL4 [48] , Pburs-GAL4 [48] , Mip 6.0 -GAL80 [48] , Kinin (drosokinin)-GAL4 [26] , Mip-GAL4 [26] , Mip 126 , UAS-Mip [26] , UAS-dTrpA1 [25] , UAS-Shi ts [24] , UAS-SPR-IR [8] , UAS-SPR [8] , UAS > stop > Shi ts [49] , UAS > stop > dTrpA1 [50] , fru FLP [51] , UAS > stop > mCD8GFP [51] , UAS > stop > nSybGFP [51] , UAS > stop > Dscam17.1-GFP [51] , dsx FLP [21] UAS > s top > Kir2.1 (a gift from Barry J. Dickson, Janelia Research Campus), LexAOP-Kir2.1 [12] , SPSN-GAL4 (VT3280-GAL4) [12] , SPSN-LexA (VT3280-LexA) [12] , SAG-GAL4 (VT50405-p65AD; VT7068-GAL4DBD) [12] , SAG-LexA (VT50405-LexA) [12] , UAS-mSP [30] , otd FLP [39] ppk-GAL4 [10] , UAS-mCD8-GFP (a gift from Barry J. Dickson, Janelia Research Campus), 189y-GAL4 (BDSC stock number, 30817), 36y-GAL4 (30819), Ddc-GAL4 (7009), Trh-GAL4 (38388), Ple-GAL4 (8848), UAS-Dicer2 (24648), Df(3 L)Exel6131 (7610), Elav-GAL4 (8760), Df(1)Exel6234 (7708), UAS-mCD8::RFP, LexAop2-mCD8::GFP;nSyb-MKII::nlsLexADBDo;UAS-p65AD::CaM (61679), hsFLP122 (1929), and Tub > GAL80 > (38879). Other stocks are generated in this study (see below). Molecular biology Amn-GAL4 , CCHa1-GAL4 , dilp7-GAL4 , Dms-GAL4 , Nplp2-GAL4 and Nplp4-GAL4 were prepared in pAGAL4, and Mip 6.0 -GAL4, Mip A -GAL4 , Mip B -GAL4 , Mip C -GAL4 and Mip D -GAL4 were prepared in the gateway vectors as described previously [52] . The GAL4 transgene was inserted into a specific site of second chromosome (VIE-72A, a gift from Barry J. Dickson, Janelia Research Campus) using ΦC31 system [53] . pAGAL4 is prepared by inserting a site-specific integration site (attB) into 7–74 site of pPTGAL4(+) vector [54] . Genomic fragments and primer sequences used to generate these are as follows: Amn-GAL4 (−3493 to +132; tatagcggccgc tttcggtgggaagttagtgc , gcgcgctctaga tgtacatataggcccgtcgtc ), CCHa1-GAL4 (−619 to +180; tatagcggccgc ttctgcctgctatgacgttg , gcgcgctctaga cgctctacctcaacacggtct ), dilp7-GAL4 (−1181 to +35; tatagcggccgc gccaggcaaataaattcagc , gcgcgctctaga cagctgcccgagttttgtat ), Dms-GAL4 (−2044 to +96; tatagcggccgc tcttctcactgcattagtcacg , gcgcgctctaga gcatagaggtggaccctgaa ), Nplp2-GAL4 (−1446 to +12; tatagcggccgc cagcatcgcacttcacattt , gcgcgctctaga gagcttggccatttttgtgt ), Nplp4-GAL4 (−832 to +149; tatagcggccgc gccggaatagaagtcgatga , gcgcgctctaga aaccagctgggaaaggaaaa ), Mip A -GAL4 (−5928 to −4626; caccagcagcaaaaagtcggaaaa, gagttcgtccatccaggaga), Mip B -GAL4 (−4626 to −3136; cacctctcctggatggacgaactc, gaaaaggctggctttgtctg), Mip C -GAL4 (−3134 to −1468; caccgacaaagccagccttttcaa, cccaaaacttgcctacaacc), and Mip D -GAL4 (-1521 to +51; caccgggatggttgtaggcaagtt, gaggagcaccatcagaaagc). Behaviour assays For behaviour assays, we followed procedures described previously [8] . Virgin males and females were collected at eclosion. Males were aged individually for 5 days; females were aged for 3 days in groups of 15–18. All assays were performed at zeitgeber time (ZT) 6:00–12:00, and repeated on at least two different days. For the mating assay, single virgin females and naive CS males were paired in 10-mm diameter chambers and videotaped (SONY DCR-SR47) for 1 h. The females that copulated were then transferred individually to food vials for 48 h. For the re-mating assay, the mated females were re-tested in the same manner with naive CS males. For rejection behaviours, either single virgin or mated females were paired with naive CS males, videotaped for 10 min at higher magnification and scored manually for ovipositor extrusions. Egg laying assays were performed in vials containing 1.5 ml of standard fly media. Virgin females were transferred to vials in groups of five for the virgin egg laying assay, and mated females were individually moved to vials for the mated egg laying assays. They were allowed to lay eggs for 48 h. The eggs laid from five virgins or one copulated female were manually counted using a stereromicroscope (ZEISS Stemi DV4). Immunohistochemistry Unless stated otherwise, 3–5-day-old virgin female or male flies were dissected under phosphate-buffered saline (PBS; pH 7.4). Tissues were fixed for 30 min at room temperature in 4% paraformaldehyde in PBS. After extensive washing, the tissues were incubated in primary antibody for 48 h at 4 °C and in secondary antibody for 24 h at 4 °C. Antibodies used were: rabbit anti-GFP (1:1000; Invitrogen, A11122), mouse anti-GFP (1:1000; Sigma, G6539), rabbit anti-DsRed (1:1000; Clontech, 632496), mouse anti-nc82 (1:50; Developmental Studies Hybridoma Bank), Alexa 488-conjugated goat anti-mouse (1:1000; Invitrogen, A11001), Alexa 488-conjugated goat anti-rabbit (1:1000; Invitrogen, A11008), Alexa 568-conjugated goat anti-mouse (1:1000; Invitrogen, A11004), and Alexa 568-conjugated goat anti-rabbit (1:1000; Invitrogen, A11011). The CNS was mounted in Vectashield (Vector Laboratory, H-1000). Images were acquired with Zeiss LSM 700/Axiovert 200 M (Zeiss), and were processed in Image J [55] . TRIC analysis Mip-GAL4 or SAG-GAL4 (VT50405-p65AD; VT7068-GAL4DBD) flies were crossed with a TRIC line (BDSC stock number, 61679; see above) to quantify the postmating changes in intracellular Ca 2+ levels in vAM and l-vPM or SAG neurons, respectively. CNS tissues from 5-day-old virgin or mated females (2 days after copulation) were processed for anti-EGFP staining as described above (see Immunohistochemistry section). To quantify EGFP fluorescence, maximum intensity Z -projections of three consecutive confocal stacks (3.82 μm-thick each) covering the entire soma of each neuron were merged with Image J. Then the relative GFP intensity of each soma was calculated by setting the average of the somas in each group from virgin females as 100%. Mosaic analysis For the mosaic analysis, we followed the procedure described in Gordon and Scott [41] with minor modifications. To generate small numbers of GAL80-negative cells, flies of the genotype tub > GAL80 > ; Mip-GAL4/UAS-dTrpA1;hs-FLP/UAS-dsRed were raised at 23 °C and subjected to a brief (~ 35 min) heat shock at 37 °C. The mosaic females were collected shortly after eclosion and aged for 3 days in groups of ~ 10. Each virgin female was then mated with naive CS males individually at 23 °C, and the mated females were kept in a single vial for 2 days. For the second mating assays, the mated mosaic females were paired with naive CS males at 30 °C for 1 h. Mosaics were separated into two groups: re-mating and non-re-mating. Induction of FLP expression earlier in development resulted in more mosaic flies with the re-mating phenotype, yet many more neurons expressing dsRed. To achieve maximally restricted labelling, FLP expression was induced at the late pupal stage (10 days after egg laying). With this protocol, the re-mating phenotype was observed in approximately 20–30% of mosaics, approximately ~ 25% more than those without FLP induction. To assess identities of activated neurons (presumably expressing both dTrpA1 and DsRed), the CNS was dissected, fixed and mounted for inspection of DsRed-expressing neurons as described in the Immunohistochemistry section. 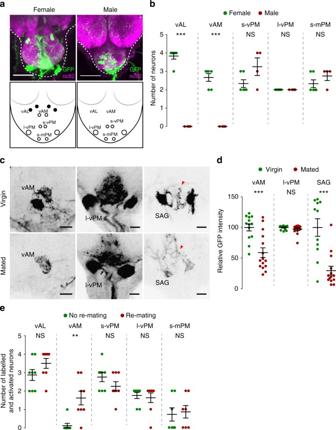Fig. 5 Sexually dimorphicMipneurons in the AG that regulate female receptivity.aMipneurons in the AG from a female (above left) and a male (above right) carryingMip-GAL4,Mip6.0-GAL80andUAS-mCD8-GFPstained by anti-GFP (green) and anti-nc82 (magenta) antibodies. The lower panels indicate the numbers and relative locations ofMipneuron somas in female (left) and male (right) AGs. TheMipneurons in the AG are grouped into six subsets: medial anterior lateral (mAL), ventral anterior lateral (vAL), ventral anterior medial (vAM), small ventral posterior medial (s-vPM), large ventral posterior medial (l-vPM), and small medial posterior medial (s-mPM). Filled and open circles indicate neurons positive and negative for anti-Mip, repectively. Scale bars, 50 μm.bThe numbers of GFP-positiveMipneurons in the AGs of females (green) and males (red) carryingMip-GAL4,Mip6.0-GAL80andUAS-mCD8-EGFP. Note the clear sexual dimorphism in thevALandvAMneurons.cNegative images of TRIC labelling (anti-GFP) in the AGs of virgin (upper panels) and mated females (lower panels), indicating intracellular Ca2+transients. Scale bars, 10 μm.dThe GFP intensities fromvAM,l-vPMandSAGneurons of TRIC females show Ca2+activity in virgin (green) and mated females (red).eThe frequencies of labelled (and therefore activated) neurons in the indicatedMipneuron subset of the AG from non-re-mating (green) and re-mating mosaic females (red). We used females carryinghsFLP,Mip-GAL4,UAS-TrpA1,UAS-DsRedandTub FRT GAL80 FRTfor stochastic manipulation (for details, see the text). NS indicates non-significance (P> 0.05); **P< 0.01, ***P< 0.001. Unpairedt-test forb,d,e. Error bars indicate s.e.m. 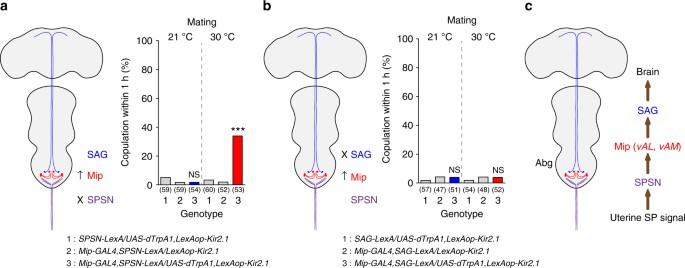Fig. 6 Mipneurons positioned within the SPSN and SAG signalling axis.a,bMating frequencies of virgin females of the indicated genotypes, scored as the percentage of females that copulate within 1 h. The numbers in parentheses indicaten. NS indicates non-significance (P> 0.05); ***P< 0.001 for comparisons against both controls (grey bars); Chi-square testa,b.cModel explaining the hierarchical relationships of the various components of the AG circuits that control female receptivity (for details, see the text) Statistical analysis Statistical analyses were performed using Prism (GraphPad Software). Data availability The authors declare that all data supporting the findings of this study are available within the paper and its Supplementary Information files.